Polarization-dependent optomechanics mediated by chiral microresonators Chirality is one of the most prominent and intriguing aspects of nature, from spiral galaxies down to aminoacids. Despite the wide range of living and non-living, natural and artificial chiral systems at different scales, the origin of chirality-induced phenomena is often puzzling. Here we assess the onset of chiral optomechanics, exploiting the control of the interaction between chiral entities. We perform an experimental and theoretical investigation of the simultaneous optical trapping and rotation of spherulite-like chiral microparticles. Due to their shell structure (Bragg dielectric resonator), the microparticles function as omnidirectional chiral mirrors yielding highly polarization-dependent optomechanical effects. The coupling of linear and angular momentum, mediated by the optical polarization and the microparticles chiral reflectance, allows for fine tuning of chirality-induced optical forces and torques. This offers tools for optomechanics, optical sorting and sensing and optofluidics. Chirality is a property connected to the lack of mirror symmetry [1] . It is a key feature in nature and has a fundamental role in several phenomena [2] . Molecules that cannot be superimposed upon their mirror images are chiral, and life has a preference for these configurations [3] , [4] . Chirality distinguishes between left- and right-handed materials, and often advances in materials science, including nanostructured materials and metamaterials, make evidence of the added value introduced by the presence of this property [5] , [6] , [7] . Circularly polarized (CP) light is another example of a chiral entity [8] . Its interaction with optically active systems enables detection of their chirality making them distinguishable through different effects [4] , [6] , [7] . This interaction suggests a methodological approach to distinguish, to measure, and also to explore chirality-related phenomena (mechanical, optical, and so on). The interaction of chiral light with achiral objects has received much interest in the field of optical trapping and manipulation, leading to a high level of optomechanical control and detection at the micro and nanoscale [9] , [10] , [11] , [12] , [13] . The observation that light can transfer spin angular momentum (SAM) to matter dates back to the pioneering work by Beth [14] in 1936, who demonstrated that CP light exerts a torque on a birefringent wave plate. From quantum mechanics, CP light with angular frequency ω carries both linear momentum (LM), ħ ω/ c , and SAM, σ ± ħ , per photon with σ + =+1 or σ − =−1 for left- or right-handed CP, respectively [14] . The development of optical tweezers [15] (OT) stimulated the exploitation of optical forces and torques in several diverse areas such as biophysics [16] , nanotechnology [13] , complex fluids [17] , [18] , [19] , [20] , [21] , microrheology [10] , [11] and microfluidics [22] , [23] . In particular, several methods have been used to induce optically controlled rotations and alignment: anisotropic scattering due to particle shape [24] , [25] , form birefringence of anisotropic objects [26] , [27] , [28] , optical birefringence [9] , [12] , [29] and transfer of angular momentum (AM) from laser beams carrying SAM and/or orbital angular momentum [12] , [30] , [31] . In optical manipulation experiments, the radiation forces and torques exerted by a CP beam are generally decoupled. However, recent experiments involving chiral particles have demonstrated the occurrence of spin-dependent radiation forces, opening a route for chiral optomechanics [32] , [33] . In this work, we measure optical trapping forces and torques on left-handed ( L -)chiral solid microparticles. We show how their broken symmetry, allowing selective reflection of CP light, is responsible for spin-dependent optomechanical effects. We optically trap spherical, non-absorbing, spherulite-like solid microparticles obtained by photopolymerization of cholesteric liquid crystal (CLC) droplets [34] . In contrast to non-polymerized CLC droplets [17] , [18] , [20] , [21] , which present significant complications due to the interaction of a strong light field with the structure of the CLC inside the droplet (for example, director distortions), the solid state of our microparticles is the key enabling feature for the observation of chiral optomechanics. Having a shell structure of refractive index connected to the helicoidal supramolecular architecture, they exhibit a selective Bragg phenomenon that makes them behave as omnidirectional chiral spherical reflectors. In contrast to conventional reflecting particles, these chiral reflectors can be set in rotation because of the transfer of SAM from light to the particle. Due to the spin-dependent selective reflection, only AM transfer from the spin component parallel to the chiral supramolecular arrangement is possible. We investigate the optomechanical effects at the birth of the photonic structure, that is, for particle radius close to the inner helical pitch. Correlation function analysis of the particle dynamics in the trap is used to measure spin-dependent trapping forces and torques originating from the coupling between the transferred LM and AM. From the ratio between the transverse trapping force constants of the two light spin states and rotation frequency measurements, we infer the onset of chirality-controlled photonic effects that occur for a specific ratio between the particle radius and the inner helical pitch. Chiral mirrors and AM transfer Consider a left-handed CP beam, with power P and angular frequency ω, that impinges on a flat partially reflecting mirror, with reflectance R and transmittance T ( Fig. 1a ). At normal incidence, the optical field undergoes a π phase-shift upon reflection, leaving its rotation sense unchanged with respect to the propagation axis. However, the propagation direction is reversed, yielding a right-handed CP reflected beam. Hence, the AM of the reflected beam is the same as the one of the incident beam. Thus, no AM is transferred to the mirror, that is, the radiation torque is zero [35] , Γ rad =0. Instead, conservation of LM yields a radiation force directed as the incident beam propagation direction and having a modulus ( Fig. 1a ). 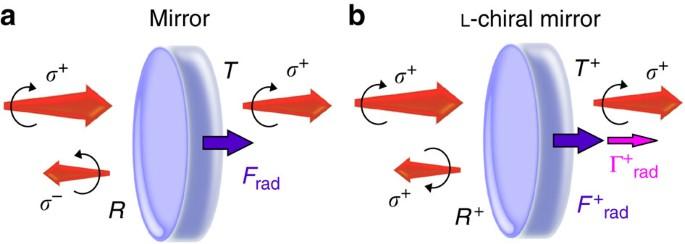Figure 1: Standard and chiral optomechanics. (a) Standard optomechanics. A CP beam of powerP, partially reflected by a conventional mirror with reflectanceR, exerts a radiation forceFrad=2RP/cand no torque on the mirror, independently on its spin state. (b) Chiral optomechanics. A left-handed CP (σ+) beam of powerP, partially reflected with reflectanceR+by a left-handed (L-) chiral mirror, exerts a radiation forceand a torqueon the mirror. Instead, the opposite spin component, σ−, is fully transmitted and has no optomechanical interaction with theL-chiral mirror. Figure 1: Standard and chiral optomechanics. ( a ) Standard optomechanics. A CP beam of power P , partially reflected by a conventional mirror with reflectance R , exerts a radiation force F rad =2RP/c and no torque on the mirror, independently on its spin state. ( b ) Chiral optomechanics. A left-handed CP (σ + ) beam of power P , partially reflected with reflectance R + by a left-handed ( L -) chiral mirror, exerts a radiation force and a torque on the mirror. Instead, the opposite spin component, σ − , is fully transmitted and has no optomechanical interaction with the L -chiral mirror. Full size image Chiral mirrors [36] have been developed employing chiral materials such as CLC [37] , [38] , [39] to provide an additional degree of freedom for the design processes via the chirality parameter. Such mirrors work differently from standard ones as they display circular Bragg reflection, that is, CP light having the same handedness of the chiral arrangement (parallel spin) and wavelength inside a specific photonic band gap is reflected, maintaining its spin state unchanged, while light having opposite handedness (antiparallel spin) is transmitted unaffected [37] , [38] . This feature allows the transfer of SAM upon reflection from the chiral mirror. In the case of a L -chiral mirror ( Fig. 1b ), a left circularly polarized (LCP) beam experiences Bragg reflection with reflectance R + , and the light polarization state is not modified upon reflection. From the conservation of LM and AM, we find the radiation force and torque on the L -chiral mirror as: Conversely, right circularly polarized (RCP) light is fully transmitted, and the radiation force and torque on the L -chiral mirror vanish, and . In the general case of elliptically polarized light the optical torque takes the form , where ϕ is the ellipticity angle ( Supplementary Note 1 ). Hence, we see that Γ rad ≥0, and vanishes for the spin state of light antiparallel to the chirality of the mirror, and thus that a radiation torque through transfer of SAM can occur even for light carrying no net SAM, that is, linear polarization. This effect can be exclusively accounted for by the broken symmetry in the interaction of the light with the chiral mirror. For a right-handed ( R -) chiral mirror, the equivalent relations depending on R − and σ − are found. Chiral microparticles Optical trapping experiments are conducted using spherical polymeric particles with a spherulite-like arrangement in which the inner structure consists of supramolecular helices originating from the centre, named radial configuration (see Fig. 2 ). The methodological approach used for the L -chiral micro-particles preparation (see Methods) is such that the helical arrangement self-organizes in precursor CLC droplets, where the helical pitch can be properly adjusted from nanometre to micrometre range by means of the chiral dopant concentration. In the CLC phase, chirality is present at the supramolecular level. In fact, the molecular director spontaneously twists about a direction perpendicular to the long molecular axis with a pitch, p , defined as the distance over which the director rotates 2π [37] , [38] . This helicoidal arrangement leads to Bragg reflection for light propagating along the helical axis and wavelength within the stop band ( Fig. 2b ). A reflectance of 100% of the light with parallel spin can be reached for a CLC slab having thickness larger than a few cholesteric pitches (see Fig. 2a ). For proper light spin and wavelength range, chiral particles with a radial configuration ( Fig. 2c–e ) behave as Bragg onion-like microresonators [40] , [41] and exhibit omnidirectional reflection, that is, they are spherical chiral microreflectors. Exploiting the above-described features, the reflectance and transmittance of these microparticles at a given wavelength can be finely controlled by tuning the light spin and the particle size (radius R 0 ). 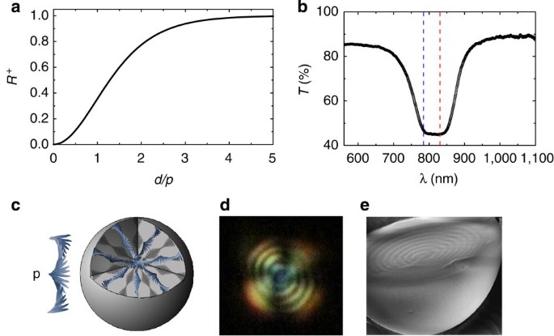Figure 2: Chiral microresonators. (a) Calculated reflection,R+, from anL-chiral layer with pitch,p, and variable thickness,d(equation 4). A reflectance close to 100% (R+≈1) is obtained for a layer thickness larger than ≈5p. (b) Measured transmission spectrum of a 20 μm-thick polymerized CLC film between two glass substrates with planar texture for linearly polarized light. The photonic band gap is centred at ≈815 nm and has a width of ≈72 nm. The dashed lines falling within the stop band are the trapping wavelengths used in the optical trapping experiments. (c) Sketch of a polymeric particle with spherulite-like (radial) configuration of the helical structure. (d) Optical microscope image of the particle between crossed polarizers: the light and dark concentric shells are due to the spatial variation of the refractive index due to the chiral structure in the radial direction. (e) Scanning electron microscope image of a half particle showing the ‘onion-like’ structure. Figure 2: Chiral microresonators. ( a ) Calculated reflection, R + , from an L -chiral layer with pitch, p , and variable thickness, d (equation 4). A reflectance close to 100% ( R + ≈1) is obtained for a layer thickness larger than ≈5 p . ( b ) Measured transmission spectrum of a 20 μm-thick polymerized CLC film between two glass substrates with planar texture for linearly polarized light. The photonic band gap is centred at ≈815 nm and has a width of ≈72 nm. The dashed lines falling within the stop band are the trapping wavelengths used in the optical trapping experiments. ( c ) Sketch of a polymeric particle with spherulite-like (radial) configuration of the helical structure. ( d ) Optical microscope image of the particle between crossed polarizers: the light and dark concentric shells are due to the spatial variation of the refractive index due to the chiral structure in the radial direction. ( e ) Scanning electron microscope image of a half particle showing the ‘onion-like’ structure. Full size image We have investigated the onset of the spin-dependent optomechanics on L -chiral particles whose radius ranges within 1–5 μm. Optomechanics with CPL and onset of the photonic effects Optical trapping is carried out in two different experimental setups with laser sources at different wavelengths, λ=830 nm and λ=785 nm, both of them fulfilling the selective reflection condition ( Fig. 2b ). The optical forces and torques on trapped particles are measured by detecting the thermal fluctuations and light-induced rotations in the effective harmonic potential by back focal plane interferometry on a quadrant photodiode (QPD; see Fig. 3a ). The particle-tracking signals are then processed by correlation function analysis [25] ( Fig. 3c ). The autocorrelation functions (ACFs) of the signals give a full account of the particle motion in the optical trap containing information on both thermal centre-of-mass positional fluctuations and rotations. Thermal positional fluctuations of the trapped particle are described by a Langevin equation [42] and yield a single exponential decay in the ACFs. Moreover, rotations about the laser beam propagation ( z -)axis are manifested in the transverse ( x,y ) fluctuating signals on the QPD, yielding a cosinusoidal modulation in the transverse ACFs [25] . 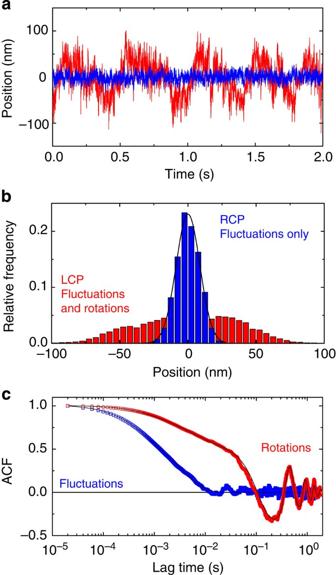Figure 3: Transverse tracking signals. (a) Transverse tracking signals for a chiral particle trapped with σ−(blue) and σ+(red) light. Rotations show up as an oscillation on top of the thermal fluctuations. (b) Histograms of the transverse position tracking. Rotations broaden the position histogram (red) deviating from the typical Gaussian profile due to thermal fluctuations (blue). (c) ACFs of particle transverse position fluctuations under σ−(blue) and σ+(red) polarizations. When the particle is not rotating (blue) a typical exponential decay is fitted to obtain the optical force constants in the OT. However, when the particle is rotating (red) signals are fitted by a superposition of an exponential, yielding the trap force constants, and an oscillation, yielding the rotation frequency (equation 3). Thus, we have for the ACF: Figure 3: Transverse tracking signals. ( a ) Transverse tracking signals for a chiral particle trapped with σ − (blue) and σ + (red) light. Rotations show up as an oscillation on top of the thermal fluctuations. ( b ) Histograms of the transverse position tracking. Rotations broaden the position histogram (red) deviating from the typical Gaussian profile due to thermal fluctuations (blue). ( c ) ACFs of particle transverse position fluctuations under σ − (blue) and σ + (red) polarizations. When the particle is not rotating (blue) a typical exponential decay is fitted to obtain the optical force constants in the OT. However, when the particle is rotating (red) signals are fitted by a superposition of an exponential, yielding the trap force constants, and an oscillation, yielding the rotation frequency (equation 3). Full size image where ω i =k i /γ( i=x,y ) are relaxation frequencies related to the trap spring constants k i and viscous translational damping γ=6πη R 0 , with η=1.002 mPas for water at 20 °C. The dynamics of about 20 different microparticles, trapped by RCP and LCP light, have been investigated as a function of their size. We observe that for RCP light, the particles are always trapped independently of their size and do not rotate. When the polarization state of the trap is switched to LCP, a size-dependent behaviour occurs. In particular, the particles with R 0 >2 μm are expelled from the trap; when R 0 <1 μm, they are trapped and do not rotate. For 1 μm <R 0 <2 μm, the microparticles are trapped and simultaneously rotate. Thus, depending on the particle size, two main phenomena originate from the interaction between chiral particles and the light carrying SAM. The first is related to the optical forces, that can be attractive or repulsive depending on the light spin state, so that larger particles may be expelled from the optical trap with parallel spin [33] , [34] . The second is related to the optical torque that originates from chirality-mediated transfer of SAM. Figure 3 shows the transverse tracking signals (a), the average position (b) and the signal ACFs (c) for a particle with radius R 0 ~1.3 μm trapped by a LCP (red) and a RCP (blue) beam. In addition to the Brownian fluctuations observed for RCP, the tracking signal ( Fig. 3a ) for LCP exhibits an oscillatory behaviour indicating that the trapped particle rotates [25] . Correspondingly ( Fig. 3b ), the histogram of the particle position has a distribution (red) much broader than the Gaussian distribution (blue) observed for RCP, resulting only from thermal positional fluctuations in the trap. To quantitatively investigate the above-described scenario, we use the transverse force constant measurements as a probe of the chiral optomechanics in the optical trap. Thus, we acquire five tracking signals for each trapped particle and each polarization state, averaging the results on all measurements made for each particle. In particular, by applying ACFs analysis ( Fig. 3c ) to each tracking signal, we get the transverse optical force constants for each spin state, k + and k − . Thus, the change in the averaged transverse force constant, , is obtained as a function of particle radius. For rotating particles, the fit of ACFs with equation 3 gives a direct measurement of the particle rotational frequency, Ω, which is used to evaluate the averaged optical torque transferred to the trapped particle. As Ω is set by the equilibrium between optical and rotational drag torques [43] , the optical torque modulus, , is equal to the rotational drag torque on a sphere rotating in a fluid at low Reynolds number [10] , . Note that we also monitor the particle dynamics in the trap by video microscopy ( Supplementary Movies 1 and 2 ) so that we can verify the absence of tumbling and the uniform rotation about the light propagation ( z − ) axis. 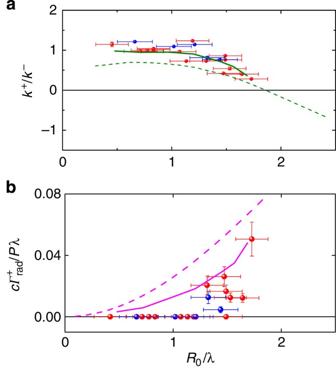Figure 4: Onset of chiral optomechanics. The occurrence of chiral optomechanical effects can be traced by looking at (a) the ratio, k+/k−, of the spin-dependent force constants and (b) the measured radiation torque, Γ+radin adimensional units as a function of the particle radius,R0, normalized to the trapping wavelength, λ. Error bars represent the standard deviation from the average value obtained for each particle data set. The green lines in (a) are calculations obtained by ray optics (dashed green line) and exact T-matrix (solid green line) modeling of optical forces on spherical particles. In (b) the dashed magenta line describes the optical torque transferred by LCP light to anL-chiral flat mirror in terms of its selective reflectivity,R+(equations 2 and 4). The solid magenta line represents T-matrix calculations of the optical torque transferred by LCP light to anL-chiral spherical particle. Figure 4a shows the ratio k + / k − as a function of the particle radius normalized to the trapping wavelength. This gives a direct evidence of the coupling between spin and optical trapping forces. In fact, as the particle radius grows and the selective reflectance increases, the trapping force constants k + lowers with respect to k − due to the consequent increase of the scattering force. In particular, for particles with R 0 /λ<1 (corresponding to R 0 <1.6 p ), the chiral structure is just formed or even absent. Thus, the reflectivity R + is negligible ( Fig. 2a ) and we expect the trapping forces to be independent of the light spin state, that is, k + ≅ k − . On the contrary, when the particle radius grows so that enough chiral layers are formed with a spherulite configuration, photonic effects become relevant and the net optical trapping force exerted by the LCP beam is lower than the one with opposite spin. In fact, in the former case, a portion of the impinging power is selectively reflected increasing the detrimental effect of the radiation pressure on the trapping itself. Thus, the force constant degeneracy is lifted and k + < k − . In the limit case of a perfect chiral photonic structure ( R + =1, T + =0), the total optical force of LCP light field becomes negative because only the radiation pressure due to the reflected light is present. Trapping of such particles with LCP light beam is not possible. Being radially symmetric, the trapped spherulite-like particles do not have macroscopic optical anisotropy [33] . Thus, transmitted light transfers only LM, and AM transfer occurs by the light reflected from the L -chiral microparticles. This in turn causes a torque on the particle itself, yielding a stable rotation. Moreover, the effect can occur only if the total LM exchanged preserves the trapping action of the light beam. The size scaling of the ratio k + / k − ( Fig. 4a ) and the radiation torque ( Fig. 4b ) displays this behaviour, that is, the onset of spin-dependent optomechanics starts to occur at R 0 /λ~1.3 ( R 0 ~2 p ). When R 0 /λ>2 ( R 0 >3 p ), the particles are rejected from the trap [33] . The data have been normalized to the different powers and the different wavelengths used in the experiments. The scaling shows how the optical torque is only related to the chiral photonic properties of the particles. As chirality is a symmetry property, the same physics remains valid for any parameter range. Figure 4: Onset of chiral optomechanics. The occurrence of chiral optomechanical effects can be traced by looking at ( a ) the ratio, k + /k − , of the spin-dependent force constants and ( b ) the measured radiation torque, Γ + rad in adimensional units as a function of the particle radius, R 0 , normalized to the trapping wavelength, λ. Error bars represent the standard deviation from the average value obtained for each particle data set. The green lines in ( a ) are calculations obtained by ray optics (dashed green line) and exact T-matrix (solid green line) modeling of optical forces on spherical particles. In ( b ) the dashed magenta line describes the optical torque transferred by LCP light to an L -chiral flat mirror in terms of its selective reflectivity, R + (equations 2 and 4). The solid magenta line represents T-matrix calculations of the optical torque transferred by LCP light to an L -chiral spherical particle. Full size image To account for the observed trapping behaviour of L -chiral microparticles, we model optical trapping forces in our experiments using both a ray optics approach [44] and exact electromagnetic calculations based on the use of the Maxwell stress tensor and electromagnetic scattering theory in the T-matrix formalism [45] , [46] , [47] . The chiral polymer refractive indices, n || and n ⊥ , at each trapping wavelength are evaluated by the Cauchy formula [33] . In the case of LCP light, the Fresnel reflection coefficient ( Fig. 2 ) near the centre of the stop band strongly depends on the effective thickness of the chiral polymer layer [33] , d , so that the reflectance is: where The reflectance R + reaches a value of about 99% for a value of d ≈5 p . However, the presence of a radial defect (S=2) [40] , going from the centre to the surface of the CLC particle, breaks the photonic structure. As a consequence, the thickness we need to consider to correctly model the photonic effects is close to R 0 . In addition, a form factor of 2/3, related to the spherical shape, must be also considered. Thus, R + for the radial particles is evaluated by using an effective thickness d =(2/3) R 0 in equation 4. Correspondingly, the transmittance T + is calculated from T + =1−R + , as the absorption of the material at the considered wavelengths is negligible. In the case of RCP illumination, the reflectance is negligible and the light is completely transmitted. These values of reflectance and transmittance have been used in the ray optics approach ( Supplementary Figs 1 and 2 , Supplementary Note 2 ) to calculate optical forces on the chiral particles, while the spring constants k + and k − are evaluated from the slope of the trapping gradient force at the equilibrium position. The result of the modelling is shown as the green dashed line in Fig. 4a . Ray optics describes the main qualitative feature of the phenomenon, that is, the light spin dependence of the optical forces connected to the microparticle chiral structure. The agreement between experiments and ray optics calculations is good for R 0 /λ>1.3. For R 0 /λ<1.3, the theoretical curve deviates from the experimental data that, on the other hand, are consistent with the assumption k + = k − . This degeneracy for small particle is expected as the particle internal structure is no longer onion-like and this prevents the photonic effects from occurring. Hence, in this regime, the optical force does not depend on the light spin but only on the light power. The discrepancy between experiment and ray optics theory can be accounted for by the limits of the validity of this approach for particles of the size considered here [48] . Indeed, ray optics is generally applicable when the particle size parameter ξ=2π R 0 /λ is much larger than one. In our measurements, ξ ranges from 3 to 10, thus in the small size regime the validity of ray optics can be questionable [48] . In order to have a quantitative description of the experimental results, we therefore developed an exact model of optical forces based on the use of the Maxwell stress tensor and electromagnetic scattering theory in the T-matrix formalism [45] , [46] , [47] ( Supplementary Fig. 3 and Supplementary Note 3 ). The exact experimental conditions (objective lens, wavelength, polarization, intensity and so on) are modelled so that the incident optical fields in the focal spot of the microscope objective are obtained in the angular spectrum representation [45] . Thus, electromagnetic scattering theory in the T-matrix formalism is applied to homogeneous dielectric particles with a real refractive index, , for RCP illumination and to partially reflecting microresonators, modelled as core-shell particles [46] , for LCP illumination. In the latter case, the core has a real refractive index , while the reflecting properties of the chiral microresonators are embedded in the thin shell that has a complex size-dependent refractive index, n shell = n ( R 0 )[1+ i α], that is needed to model the size-dependent reflectance (based on equation 4) of the chiral particles ( Supplementary Note 3 ). The T-matrix calculations are shown as the green solid line in Fig. 4a . Their quantitative agreement with experiments is excellent, showing strikingly that optical forces on chiral microparticles are a consequence of the partial reflection related to the Bragg chiral structure formation. In Fig. 4b , the measured optical torque transferred by LCP light to the L -chiral microparticles is first compared with the optical torque exerted on a flat L -chiral mirror (dashed magenta line) calculated using equations 2 and 4 in terms of its selective reflectivity, R + . This represents the maximum optical torque that can be transferred upon reflection of LCP light and, as expected, the experimental values are systematically lower than the calculated curve. Instead, the solid magenta line is the optical torque transferred from LCP light to the microresonators, modelled as core-shell spherical particles, and calculated using electromagnetic scattering theory [47] . Also in this case, we find a good agreement between experiments and theory as soon as we observe the L -chiral particles rotating and the chiral structure forms, that is, for R 0 /λ>1.3. In conclusion, we have reported an experimental investigation of polarization-dependent optical forces and torques on chiral microparticles working as omnidirectional chiral microresonators. The inner Bragg onion structure of the particle and the correspondent selective reflection for light wavelength in the stop band, allows SAM transfer only from the light component having spin parallel to the particle handedness. We have observed optomechanical effects originating from the coupling of transferred LM and AM mediated by the particle chirality. We have shown simultaneous optical trapping and rotation connected to light spin selective reflection exhibited by the chiral particles, and their control by means of the particle reflectance and light spin. Chirality-controlled optical trapping and manipulation can be exploited to address novel strategies for optomechanics experiments and optical sorting [49] . Furthermore, spin-dependent optical forces pave the way to novel methodologies for optical cooling and trapping based on the coupling of translational and rotational degrees of freedom towards the quantum mechanical motional ground states of levitated particles [12] , [50] , [51] , [52] . For L -chiral microparticles, the centre-of-mass and rotations could be actively laser cooled in a σ + σ + counter-propagating beams configuration. The angular degrees of freedom would be clamped by the opposite optical torque induced by the counter-propagating beams. As both radiation force and torque are dependent on intensity and polarization, a feedback cooling scheme for all degrees of freedom could be efficiently applied either by changing the light intensity or by controlling the light polarization. Finally, the method used to create chiral microparticles allows embedding resonant nanoparticles at the central defect, with prospects for microcavity optomechanics in optical traps. Preparation of the chiral particles The L -chiral microparticles are prepared through the following steps. First, a pure reactive mesogen contained in RMS03-001C blend (Merck, Germany) is obtained extracting its solvent PGMEA (propylene glycol monomethyl ether acetate) by vacuum evaporation at 90 °C. Thus, this is mixed with 14 wt% L -chiral dopant (ZLI-811, Merck) yielding a CLC phase. This has a photonic band gap centred at ≈815 nm, fulfilling the selective reflection condition for both the wavelengths, 830 and 785 nm, used in the optical trapping experiments. Then, a CLC droplet emulsion is prepared with type I ultrapure water (18.2 MΩ cm resistivity at 25°C, <5 ppb total organic carbon). The emulsion is polymerized in nitrogen environment for at least 4 h under a 2 mW cm −2 intensity UV lamp (Mega Electronics lamp mod. LV202-E) having emission wavelength centred at about 350 nm. The size of the solid chiral particles produced by this method ranges from hundreds of nanometres up to tens of microns. The resulting helicoidal pitch, p , is approximately 513 nm. Finally, a few tens of microlitres of the chiral particles suspension are loaded in a small glass chamber for OT experiments. OT setups Optical trapping is carried out in two different experimental setups. In brief, both use a near-infrared laser beam, 830 nm (150 mW) or 785 nm (80 mW), from diode laser sources. The beam is expanded to overfill a high numerical aperture objective (NA=1.3) to obtain a diffraction-limited spot. A quarter-wave plate, placed in the beam path, is used to control the light spin state. Optical force and torque on the trapped particle are measured by detecting the thermal fluctuations in the effective harmonic potential. Back focal plane interferometry, where the interference between a laser beam and the light scattered by a trapped particle is collected on a QPD (Thorlabs), is used in forward (830 nm setup) or backward (785 nm setup) detection. Data acquisition boards are used to collect the signals from the QPD through a PC. Finally, charge-coupled device cameras are used to monitor the trapped particles ( Supplementary Movies 1 and 2 ). How to cite this article: Donato, M. G. et al. Polarization-dependent optomechanics mediated by chiral microresonators. Nat. Commun. 5:3656 doi: 10.1038/ncomms4656 (2014).